Genetic correlation between amyotrophic lateral sclerosis and schizophrenia We have previously shown higher-than-expected rates of schizophrenia in relatives of patients with amyotrophic lateral sclerosis (ALS), suggesting an aetiological relationship between the diseases. Here, we investigate the genetic relationship between ALS and schizophrenia using genome-wide association study data from over 100,000 unique individuals. Using linkage disequilibrium score regression, we estimate the genetic correlation between ALS and schizophrenia to be 14.3% (7.05–21.6; P =1 × 10 −4 ) with schizophrenia polygenic risk scores explaining up to 0.12% of the variance in ALS ( P =8.4 × 10 −7 ). A modest increase in comorbidity of ALS and schizophrenia is expected given these findings (odds ratio 1.08–1.26) but this would require very large studies to observe epidemiologically. We identify five potential novel ALS-associated loci using conditional false discovery rate analysis. It is likely that shared neurobiological mechanisms between these two disorders will engender novel hypotheses in future preclinical and clinical studies. Amyotrophic lateral sclerosis (ALS) is a late-onset neurodegenerative condition characterized by progressive loss of upper and lower motor neurons, leading to death from respiratory failure in 70% of patients within 3 years of symptom onset. Although ALS is often described as a primarily motor-system disease, extramotor involvement occurs in up to 50% of cases, with prominent executive and behavioural impairment, and behavioural variant frontotemporal dementia (FTD) in up to 14% of cases [1] . A neuropsychiatric prodrome has been described in some people with ALS–FTD, and higher rates of schizophrenia and suicide have been reported in first and second degree relatives of those with ALS, particularly in kindreds associated with the C9orf72 hexanucleotide repeat expansion [2] . These clinical and epidemiological observations suggest that ALS and schizophrenia may share heritability. ALS and schizophrenia both have high heritability estimates (0.65 and 0.64, respectively) [3] , [4] ; however the underlying genetic architectures of these heritable components appear to differ. Analysis of large genome-wide association study (GWAS) datasets has implicated over 100 independent risk loci for schizophrenia [5] and estimated that a substantial proportion (23%) of the variance in underlying liability for schizophrenia is due to additive polygenic risk (many risk-increasing alleles of low individual effect combining to cause disease) conferred by common genetic variants [6] . This proportion, the single nucleotide polymorphism (SNP)-based heritability, is lower in ALS (8.2%), in which fewer than ten risk loci have been identified by GWAS [7] . Nevertheless, both diseases have polygenic components, but the extent to which they overlap has not been investigated. Recently, methods to investigate overlap between polygenic traits using GWAS data have been developed [8] , [9] , [10] . These methods assess either pleiotropy (identical genetic variants influencing both traits) or genetic correlation (identical alleles influencing both traits). Genetic correlation is related to heritability; for both measures, binary traits such as ALS and schizophrenia are typically modelled as extremes of an underlying continuous scale of liability to develop the trait. If two binary traits are genetically correlated, their liabilities covary, and this covariance is determined by both traits having identical risk alleles at overlapping risk loci. Studies of pleiotropy and genetic correlation have provided insights into the overlapping genetics of numerous traits and disorders, although none to date has implicated shared polygenic risk between neurodegenerative and neuropsychiatric disease. Here, we apply several techniques to identify and dissect the polygenic overlap between ALS and schizophrenia. We provide evidence for genetic correlation between the two disorders which is unlikely to be driven by diagnostic misclassification and we demonstrate a lack of polygenic overlap between ALS and other neuropsychiatric and neurological conditions, which could be due to limited power given the smaller cohort sizes for these studies. Genetic correlation between ALS and schizophrenia To investigate the polygenic overlap between ALS and schizophrenia, we used individual-level and summary data from GWAS for ALS [7] (36,052 individuals) and schizophrenia [5] (79,845 individuals). At least 5,582 control individuals were common to both datasets, but for some cohorts included in the schizophrenia dataset this could not be ascertained so this number is likely to be higher. For ALS, we used summary data from both mixed linear model association testing [11] and meta-analysis of cohort-level logistic regression [12] . We first used linkage disequilibrium (LD) score regression with ALS and schizophrenia summary statistics; this technique models, for polygenic traits, a linear relationship between a SNP’s LD score (the amount of genetic variation that it captures) and its GWAS test statistic [13] . This distinguishes confounding from polygenicity in GWAS inflation and the regression coefficient can be used to estimate the SNP-based heritability ( h S 2 ) for single traits [13] . In the bivariate case, the regression coefficient estimates genetic covariance ( ρ g ) for pairs of traits, from which genetic correlation ( r g ) is estimated [8] ; these estimates are unaffected by sample overlap between traits. Using constrained intercept LD score regression with mixed linear model ALS summary statistics, we estimated the liability-scale SNP-based heritability of ALS to be 8.2% (95% confidence interval=7.2–9.1; mean χ 2 =1.13; all ranges reported below indicate 95% confidence intervals), replicating previous estimates based on alternative methods [7] . 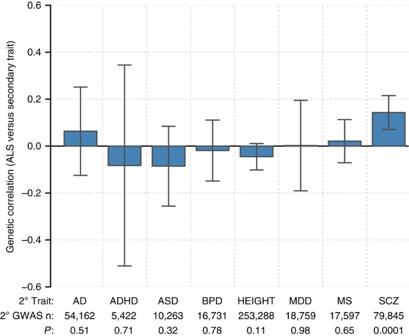Figure 1: Genetic correlation between ALS and eight secondary traits. Error bars indicating 95% confidence intervals andP-values were calculated by the LD score regression software using a block jackknife procedure. Secondary traits are: AD, Alzheimer’s disease; ADHD, attention deficit-hyperactivity disorder; ASD, autism spectrum disorder; BPD, bipolar disorder; MDD, major depressive disorder; MS, multiple sclerosis; SCZ, schizophrenia. 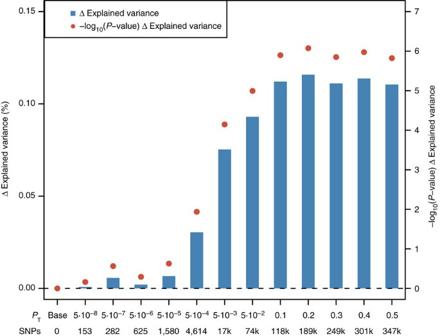Figure 2: Analysis of PRS for schizophrenia in a target sample of 10,032 ALS cases and 16,627 healthy controls. P-value thresholds (PT) for schizophrenia SNPs are shown on thexaxis, where the number of SNPs increases with a more lenientPT. Δ Explained variances (NagelkerkeR2, shown as a %) of a generalized linear model including schizophrenia-based PRS versus a baseline model without polygenic scores (blue bars) are shown for eachPT. −Log10P-values of Δ explained variance perPT(red dots) representP-values from the binomial logistic regression of ALS phenotype on PRS, accounting for LD (Supplementary Table 4) and including sex and significant principal components as covariates (Supplementary Fig. 2). Values are provided inSupplementary Table 5. Estimates based on ALS meta-analysis summary statistics and free-intercept LD score regression with mixed linear model summary statistics were lower ( Supplementary Table 1 ), resulting in higher genetic correlation estimates ( Supplementary Table 2 ); for this reason, we conservatively use constrained intercept genetic correlation estimates for ALS mixed linear model summary statistics throughout the remainder of this paper. Heritability estimates for permuted ALS data were null ( Supplementary Table 1 ). LD score regression estimated the genetic correlation between ALS and schizophrenia to be 14.3% (7.05–21.6; P =1 × 10 −4 ). Results were similar for a smaller schizophrenia cohort of European ancestry (21,856 individuals) [14] , indicating that the inclusion of individuals of Asian ancestry in the schizophrenia cohort did not bias this result ( Supplementary Fig. 1 ). In addition to schizophrenia, we estimated genetic correlation with ALS using GWAS summary statistics for bipolar disorder [15] , major depressive disorder [16] , attention deficit-hyperactivity disorder [17] , autism spectrum disorder [17] , Alzheimer's disease ( Supplementary Note 1 ) [18] , multiple sclerosis [19] and adult height [20] , finding no significant genetic correlation between ALS and any secondary trait other than schizophrenia ( Fig. 1 ; Supplementary Table 2 ). Figure 1: Genetic correlation between ALS and eight secondary traits. Error bars indicating 95% confidence intervals and P -values were calculated by the LD score regression software using a block jackknife procedure. Secondary traits are: AD, Alzheimer’s disease; ADHD, attention deficit-hyperactivity disorder; ASD, autism spectrum disorder; BPD, bipolar disorder; MDD, major depressive disorder; MS, multiple sclerosis; SCZ, schizophrenia. Full size image Polygenic risk score analysis We supported the positive genetic correlation between ALS and schizophrenia by analysis of polygenic risk for schizophrenia in the ALS cohort. Polygenic risk scores (PRS) are per-individual scores based on the sum of alleles associated with one phenotype, weighted by their effect size, measured in an independent target sample of the same or a different phenotype [10] . PRS calculated on schizophrenia GWAS summary statistics for twelve P -value thresholds ( P T ) explained up to 0.12% ( P T =0.2, P =8.4 × 10 −7 ) of the phenotypic variance in a subset of the individual-level ALS genotype data that had all individuals removed that were known or suspected to be present in the schizophrenia cohort ( Fig. 2 ; Supplementary Table 5 ). ALS cases had on average higher PRS for schizophrenia compared to healthy controls and harbouring a high schizophrenia PRS for P T =0.2 significantly increased the odds of being an ALS patient in our cohort ( Fig. 3 ; Supplementary Table 6 ). Permutation of case–control labels reduced the explained variance to values near zero ( Supplementary Fig. 3 ). Figure 2: Analysis of PRS for schizophrenia in a target sample of 10,032 ALS cases and 16,627 healthy controls. P -value thresholds ( P T ) for schizophrenia SNPs are shown on the x axis, where the number of SNPs increases with a more lenient P T . Δ Explained variances (Nagelkerke R 2 , shown as a %) of a generalized linear model including schizophrenia-based PRS versus a baseline model without polygenic scores (blue bars) are shown for each P T . −Log 10 P -values of Δ explained variance per P T (red dots) represent P -values from the binomial logistic regression of ALS phenotype on PRS, accounting for LD ( Supplementary Table 4 ) and including sex and significant principal components as covariates ( Supplementary Fig. 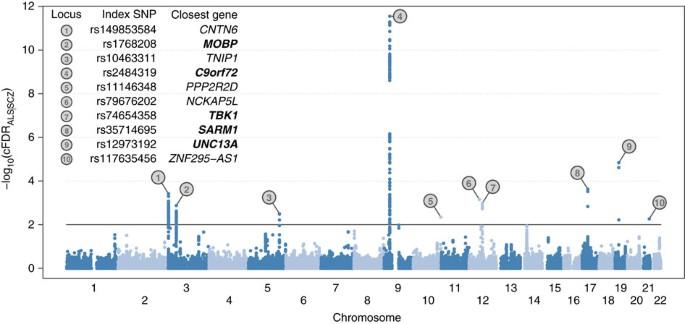Figure 4: Pleiotropy-informed ALS risk loci determined by analysis of cFDR in ALS GWASP-values given schizophrenia GWASP-values (cFDRALS|SCZ). Each point denotes a SNP; itsxaxis position corresponds to its chromosomal location and its height indicates the extent of association with ALS by cFDR analysis. The solid line indicates the threshold cFDR=0.01. Any gene whose role in ALS is already established is in bold. A complete list of all loci at cFDR⩽0.05 is provided inSupplementary Table 8. 2 ). 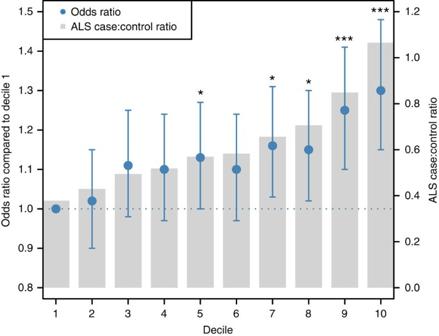Values are provided in Supplementary Table 5 . Figure 3: Odds ratio for ALS by PRS deciles for schizophrenia. The figure applies to schizophreniaP-value threshold (PT)=0.2. The PRS for this threshold were converted to ten deciles containing near identical numbers of individuals. Decile 1 contained the lowest scores and decile 10 contained the highest scores, where decile 1 was the reference and deciles 2–10 were dummy variables to contrast to decile 1 for OR calculation. The case:control ratio per decile is indicated with grey bars. Error bars indicate 95% confidence intervals. Significant differences from decile 1 were determined by logistic regression of ALS phenotype on PRS decile, including sex and principal components as covariates and are indicated by *P<0.05 or ***P<0.001. Full size image Figure 3: Odds ratio for ALS by PRS deciles for schizophrenia. The figure applies to schizophrenia P -value threshold ( P T )=0.2. The PRS for this threshold were converted to ten deciles containing near identical numbers of individuals. Decile 1 contained the lowest scores and decile 10 contained the highest scores, where decile 1 was the reference and deciles 2–10 were dummy variables to contrast to decile 1 for OR calculation. The case:control ratio per decile is indicated with grey bars. Error bars indicate 95% confidence intervals. Significant differences from decile 1 were determined by logistic regression of ALS phenotype on PRS decile, including sex and principal components as covariates and are indicated by * P <0.05 or *** P <0.001. Full size image Modelling misdiagnosis and comorbidity Using BUHMBOX [21] , a tool that distinguishes true genetic relationships between diseases (pleiotropy) from spurious relationships resulting from heterogeneous mixing of disease cohorts, we determined that misdiagnosed cases in the schizophrenia cohort (for example, young-onset FTD–ALS) did not drive the genetic correlation estimate between ALS and schizophrenia ( P =0.94). Assuming a true genetic correlation of 0%, we estimated the required rate of misdiagnosis of ALS as schizophrenia to be 4.86% (2.47–7.13) to obtain the genetic correlation estimate of 14.3% (7.05–21.6; Supplementary Table 7 ), which we consider to be too high to be likely. However, if ALS and schizophrenia are genetically correlated, more comorbidity would be expected than if the genetic correlation was 0%. Modelling our observed genetic correlation of 14.3% (7.05–21.6), we estimated the odds ratio for having above-threshold liability for ALS given above-threshold liability for schizophrenia to be 1.17 (1.08–1.26), and the same for schizophrenia given ALS ( Supplementary Fig. 4 ). From a clinical perspective, to achieve 80% power to detect a significant (α=0.05) excess of schizophrenia in the ALS cohort as a result of this genetic correlation, the required population-based incident cohort size is 16,448 ALS patients (7,310–66,670). Pleiotropic risk loci We leveraged the genetic correlation between ALS and schizophrenia to discover novel ALS-associated genomic loci by conditional false discovery rate (cFDR) analysis [9] , [22] ( Fig. 4 ; Supplementary Table 8 ). Five loci already known to be involved in ALS were identified (corresponding to MOBP , C9orf72 , TBK1 , SARM1 and UNC13A ) along with five potential novel loci at cFDR<0.01 ( CNTN6 , TNIP1 , PPP2R2D , NCKAP5L and ZNF295-AS1 ). No gene set was significantly enriched (after Bonferroni correction) in genome-wide cFDR values when analysed using MAGENTA. Figure 4: Pleiotropy-informed ALS risk loci determined by analysis of cFDR in ALS GWAS P -values given schizophrenia GWAS P -values (cFDR ALS|SCZ ). Each point denotes a SNP; its x axis position corresponds to its chromosomal location and its height indicates the extent of association with ALS by cFDR analysis. The solid line indicates the threshold cFDR=0.01. Any gene whose role in ALS is already established is in bold. A complete list of all loci at cFDR ⩽ 0.05 is provided in Supplementary Table 8 . Full size image There is evolving clinical, epidemiological and biological evidence for an association between ALS and psychotic illness, particularly schizophrenia. Genetic evidence of overlap to date has been based primarily on individual genes showing Mendelian inheritance, in particular the C9orf72 hexanucleotide repeat expansion, which is associated with ALS and FTD, and with psychosis in relatives of ALS patients [2] . In this study, we have replicated SNP-based heritability estimates for ALS and schizophrenia using GWAS summary statistics, and have for the first time demonstrated significant overlap between the polygenic components of both diseases, estimating the genetic correlation to be 14.3%. We have carefully controlled for confounding bias, including population stratification and shared control samples, and have shown through analysis of polygenic risk scores that the overlapping polygenic risk applies to SNPs that are modestly associated with both diseases. Given that our genetic correlation estimate relates to the polygenic components of ALS ( h S 2 =8.2%) and schizophrenia ( h S 2 =23%) and these estimates do not represent all heritability for both diseases, the accuracy of using schizophrenia-based PRS to predict ALS status in any patient is expected to be low (Nagelkerke’s R 2 =0.12% for P T =0.2), although statistically significant ( P =8.4 × 10 −7 ). Nevertheless, the positive genetic correlation of 14.3% indicates that the direction of effect of risk-increasing and protective alleles is consistently aligned between ALS and schizophrenia, suggesting convergent biological mechanisms between the two diseases. Although phenotypically heterogeneous, both ALS and schizophrenia are clinically recognizable as syndromes [23] , [24] . The common biological mechanisms underlying the association between the two conditions are not well understood, but are likely associated with disruption of cortical networks. Schizophrenia is a polygenic neurodevelopmental disorder characterized by a combination of positive symptoms (hallucinations and delusions), negative symptoms (diminished motivation, blunted affect, reduction in spontaneous speech and poor social functioning) and impairment over a broad range of cognitive abilities [25] . ALS is a late onset complex genetic disease characterized by a predominantly motor phenotype with recently recognized extra-motor features in 50% of patients, including cognitive impairment [1] . It has been suggested that the functional effects of risk genes in schizophrenia converge by modulating synaptic plasticity, and influencing the development and stabilization of cortical microcircuitry [5] . In this context, our identification of CNTN6 (contactin 6, also known as NB-3, a neural adhesion protein important in axon development) [26] as a novel pleiotropy-informed ALS-associated locus supports neural network dysregulation as a potential convergent mechanism of disease in ALS and schizophrenia. No significantly enriched biological pathway or ontological term was identified within genome-wide cFDR values using MAGENTA. Low inflation in ALS GWAS statistics, coupled with a rare variant genetic architecture [7] , render enrichment-based biological pathway analyses with current sample sizes challenging. Nevertheless, nine further loci were associated with ALS risk at cFDR <0.01. Of these, MOBP , C9orf72 , TBK1 , SARM1 and UNC13A have been described previously in ALS and were associated by cFDR analysis in this study owing to their strong association with ALS through GWAS [7] . The remaining four loci ( TNIP1 , PPP2R2D , NCKAP5L and ZNF295-AS1 ) are novel associations and may represent pleiotropic disease loci. TNIP1 encodes TNFAIP3 interacting protein 1 and is involved in autoimmunity and tissue homoeostasis [27] . The protein product of PPP2R2D is a regulatory subunit of protein phosphatase 2 and has a role in PI3K-Akt signalling and mitosis [28] . NCKAP5L is a homologue of NCKAP5 , encoding NAP5, a proline-rich protein that has previously been implicated in schizophrenia, bipolar disorder and autism [29] , [30] . ZNF295-AS1 is a noncoding RNA [31] . Further investigation into the biological roles of these genes may yield novel insight into the pathophysiology of certain subtypes of ALS and schizophrenia, and as whole-genome and exome datasets become available in the future for appropriately large ALS case–control cohorts, testing for burden of rare genetic variation across these genes will be particularly instructive, especially given the role that rare variants appear to play in the pathophysiology of ALS [7] . Our data suggest that other neuropsychiatric conditions (bipolar disorder, autism and major depression) do not share polygenic risk with ALS. This finding contrasts with our recent observations from family aggregation studies and may be unexpected given the extensive genetic correlation between neuropsychiatric conditions [6] . This could relate to statistical power conferred by secondary phenotype cohort sizes, and future studies with larger sample sizes will shed further light on the relationship between ALS and neuropsychiatric disease. It is also possible that the current study underestimates genetic correlations due to the substantial role that rare variants play in the genetic architecture of ALS [7] and future fine-grained studies examining heritability and genetic correlation in low-minor allele frequency and low-LD regions may identify a broader relationship between ALS and neuropsychiatric diseases. A potential criticism of this study is that the polygenic overlap between ALS and schizophrenia could be driven by misdiagnosis, particularly in cases of ALS–FTD, which can present in later life as a psychotic illness and could be misdiagnosed as schizophrenia. This is unlikely, as strict diagnostic criteria are required for inclusion of samples in the schizophrenia GWAS dataset [5] . Furthermore, since core schizophrenia symptoms are usually diagnosed during late adolescence, a misdiagnosis of FTD-onset ALS–FTD as schizophrenia is unlikely. In this study, we found no evidence for misdiagnosis of ALS as schizophrenia (BUHMBOX P =0.94) and we estimated that a misdiagnosis of 4.86% of ALS cases would be required to spuriously observe a genetic correlation of 14.3%, which is not likely to occur in clinical practice. We are therefore confident that this genetic correlation estimate reflects a genuine polygenic overlap between the two diseases and is not a feature of cohort ascertainment, but the possibility of some misdiagnosis in either cohort cannot be entirely excluded based on available data. A positive genetic correlation between ALS and schizophrenia predicts an excess of patients presenting with both diseases. Most neurologists and psychiatrists, however, will not readily acknowledge that these conditions co-occur frequently. Our genetic correlation estimate confers an odds ratio of 1.17 (1.08–1.26) for harbouring above-threshold liability for ALS given schizophrenia (or vice versa) and a lifetime risk of 1:34,336 for both phenotypes together. Thus, a very large incident cohort of 16,448 ALS patients (7,310–66,670), with detailed phenotype information, would be required to have sufficient power to detect an excess of schizophrenia within an ALS cohort. Coupled with reduced life expectancy in patients with schizophrenia [32] , this may explain the relative dearth of epidemiological studies to date providing clinical evidence of excess comorbidity. Moreover, it has also been proposed that prolonged use of antipsychotic medication may protect against developing all of the clinical features of ALS [33] , which would reduce the rate of observed comorbidity. Considering our novel evidence for a genetic relationship between ALS and schizophrenia, this underscores the intriguing possibility that therapeutic strategies for each condition may be useful in the other, and our findings provide rationale to consider the biology of ALS and schizophrenia as related in future drug development studies. Indeed, the glutamate-modulating ALS therapy riluzole has shown efficacy as an adjunct to risperidone, an antipsychotic medication, in reducing the negative symptoms of schizophrenia [34] . In conclusion, we have estimated the genetic correlation between ALS and schizophrenia to be 14.3% (7.05–21.6), providing molecular genetic support for our epidemiological observation of psychiatric endophenotypes within ALS kindreds. To our knowledge, this is the first study to show genetic correlation derived from polygenic overlap between neurodegenerative and neuropsychiatric phenotypes. The presence of both apparent monogenic C9orf72 -driven overlap [2] and polygenic overlap in the aetiology of ALS and schizophrenia suggests the presence of common biological processes, which may relate to disruption of cortical circuitry. As both ALS and schizophrenia are heterogeneous conditions, further genomic, biological and clinical studies are likely to yield novel insights into the pathological processes for both diseases and will provide clinical sub-stratification parameters that could drive novel drug development for both neurodegenerative and psychiatric conditions. Study population and genetic data For ALS, 7,740,343 SNPs genotyped in 12,577 ALS patients and 23,475 healthy controls of European ancestry organized in 27 platform- and country-defined strata were used [7] . The schizophrenia dataset comprised GWAS summary statistics for 9,444,230 SNPs originally genotyped in 34,241 patients and 45,604 controls of European and Asian ancestry [5] . For LD score regression, GWAS summary statistics were generated for the ALS cohort using mixed linear model association testing implemented in Genome-wide Complex Trait Analysis [11] or logistic regression combined with cross-stratum meta-analysis using METAL [12] . To evaluate sample overlap for PRS and cFDR analyses, we also obtained individual-level genotype data for 27,647 schizophrenia cases and 33,675 controls from the schizophrenia GWAS (Psychiatric Genomics Consortium [5] and dbGaP accession number phs000021.v3.p2). Using 88,971 LD-pruned (window size 200 SNPs; shift 20 SNPs; r 2 >0.25) SNPs in both datasets (INFO score>0.8; MAF>0.2), with SNPs in high-LD regions removed ( Supplementary Table 4 ), samples were removed from the ALS dataset if they were duplicated or had a cryptically related counterpart (PLINK >0.1; 5,582 individuals) in the schizophrenia cohort and whole strata (representing Finnish and German samples; 3,811 individuals) were also removed if commonality with the schizophrenia cohort could not be ascertained (due to unavailability of individual-level genotype data in the schizophrenia cohort) and in which a sample overlap was suspected ( Supplementary Table 3 ). LD score regression We calculated LD scores using LDSC v1.0.0 in 1 centiMorgan windows around 13,307,412 non-singleton variants genotyped in 379 European individuals (CEU, FIN, GBR, IBS and TSI populations) in the phase 1 integrated release of the 1,000 Genomes Project [35] . For regression weights [13] , we restricted LD score calculation to SNPs included in both the GWAS summary statistics and HapMap phase 3; for r g estimation in pairs of traits this was the intersection of SNPs for both traits and HapMap. Because population structure and confounding were highly controlled in the ALS summary statistics by the use of mixed linear model association tests, we constrained the LD score regression intercept to 1 for h S 2 estimation in ALS, and we also estimated h S 2 with a free intercept. For h S 2 estimation in all other traits and for r g estimation the intercept was a free parameter. We also estimated r g using ALS meta-analysis results [7] with free and constrained intercepts and with permuted data conserving population structure. Briefly, principal component analysis was carried out for each stratum using smartpca [36] and the three-dimensional space defined by principal components 1–3 was equally subdivided into 1,000 cubes. Within each cube, case–control labels were randomly swapped and association statistics were re-calculated for the entire stratum using logistic regression. Study-level P -values were then calculated using inverse variance weighted fixed effect meta-analysis implemented in METAL [7] , [12] . h S 2 was estimated for these meta-analysed permuted data using LD score regression ( Supplementary Table 1 ). Polygenic risk score analysis We calculated PRS for 10,032 cases and 16,627 healthy controls in the ALS dataset (duplicate and suspected or confirmed related samples with the schizophrenia dataset removed), based on schizophrenia-associated alleles and effect sizes reported in the GWAS summary statistics for 6,843,674 SNPs included in both studies and in the phase 1 integrated release of the 1,000 Genomes Project [35] (imputation INFO score <0.3; minor allele frequency <0.01; A/T and G/C SNPs removed). SNPs were clumped in two rounds (physical distance threshold of 250 kb and a LD threshold ( R 2 ) of>0.5 in the first round and a distance of 5,000 kb and LD threshold of >0.2 in the second round) using PLINK v1.90b3y, removing high-LD regions ( Supplementary Table 4 ), resulting in a final set of 496,548 SNPs for PRS calculations. Odds ratios for autosomal SNPs reported in the schizophrenia summary statistics were log-converted to beta values and PRS were calculated using PLINK’s score function for twelve schizophrenia GWAS P -value thresholds ( P T ): 5 × 10 −8 , 5 × 10 −7 , 5 × 10 −6 , 5 × 10 −5 , 5 × 10 −4 , 5 × 10 −3 , 0.05, 0.1, 0.2, 0.3, 0.4 and 0.5. A total of 100 principal components (PCs) were generated for the ALS sample using GCTA version 1.24.4. Using R version 3.2.2, a generalized linear model was applied to model the phenotype of individuals in the ALS dataset. PCs that had a significant effect on the phenotype ( P <0.0005, Bonferroni-corrected for 100 PCs) were selected (PCs 1, 4, 5, 7, 8, 10, 11, 12, 14, 36, 49). To estimate explained variance of PRS on the phenotype, a baseline linear relationship including only sex and significant PCs as variables was modelled first: where y is the phenotype in the ALS dataset, α is the intercept of the model with a slope β for each variable x . Subsequently, a linear model including polygenic scores for each schizophrenia P T was calculated: A Nagelkerke R 2 value was obtained for every model and the baseline Nagelkerke R 2 value was subtracted, resulting in a Δ explained variance that describes the contribution of schizophrenia-based PRS to the phenotype in the ALS dataset. PRS analysis was also performed in permuted case–control data (1,000 permutations, conserving case–control ratio) to assess whether the increased Δ explained variance was a true signal associated with phenotype. Δ explained variances and P -values were averaged across permutation analyses. To ensure we did not over- or under-correct for population effects in our model, we tested the inclusion of up to a total of 30 PCs in the model, starting with the PC with the most significant effect on the ALS phenotype ( Supplementary Fig. 2 ). Increasing the number of PCs initially had a large effect on the Δ explained variance, but this effect levelled out after 11 PCs. On the basis of this test we are confident that adding the 11 PCs that had a significant effect on the phenotype sufficiently accounted for possible confounding due to population differences. For the schizophrenia P T for which we obtained the highest Δ explained variance (0.2), we subdivided observed schizophrenia-based PRS in the ALS cohort into deciles and calculated the odds ratio for being an ALS case in each decile compared to the first decile using a similar generalized linear model: Odds ratios and 95% confidence intervals for ALS were derived by calculating the exponential function of the beta estimate of the model for each of the deciles 2–10. Diagnostic misclassification To distinguish the contribution of misdiagnosis from true genetic pleiotropy we used BUHMBOX [21] with 417 independent ALS risk alleles in a sample of 27,647 schizophrenia patients for which individual-level genotype data were available. We also estimated the required misdiagnosis rate M of FTD–ALS as schizophrenia that would lead to the observed genetic correlation estimate as C /( C +1), where C = ρ g N SCZ / N ALS and N SCZ and N ALS are the number of cases in the schizophrenia and ALS datasets, respectively [37] (derived in Supplementary Methods 1 ). Expected comorbidity To investigate the expected comorbidity of ALS and schizophrenia given the observed genetic correlation, we modelled the distribution in liability for ALS and schizophrenia as a bivariate normal distribution with the liability-scale covariance determined by LD score regression ( Supplementary Methods 2 ). Lifetime risks for ALS [38] and schizophrenia [25] of 1/400 and 1/100, respectively, were used to calculate liability thresholds above which individuals develop ALS or schizophrenia, or both. The expected proportions of individuals above these thresholds were used to calculate the odds ratio of developing ALS given schizophrenia, or vice versa ( Supplementary Methods 2 ). The required population size to observe a significant excess of comorbidity was calculated using the binomial power equation. Pleiotropy-informed risk loci for ALS Using an adapted cFDR method [9] that allows shared controls between cohorts [22] , we estimated per-SNP cFDR given LD score-corrected [8] schizophrenia GWAS P -values for ALS mixed linear model summary statistics calculated in a dataset excluding Finnish and German cohorts (in which suspected control overlap could not be determined), but including all other overlapping samples (totalling 5,582). To correct for the relationship between LD and GWAS test statistics, schizophrenia summary statistics were residualized on LD score by subtracting the product of each SNP’s LD score and the univariate LD score regression coefficient for schizophrenia. cFDR values conditioned on these residualized schizophrenia GWAS P -values were calculated for mixed linear model association statistics calculated at 6,843,670 SNPs genotyped in 10,147 ALS cases and 22,094 controls. Pleiotropic genomic loci were considered statistically significant if cFDR<0.01 (following Andreassen et al . [9] ) and were clumped with all neighbouring SNPs based on LD ( r 2 >0.1) in the complete ALS dataset. Associated cFDR genomic regions were then mapped to the locations of known RefSeq transcripts in human genome build GRCh37. Genome-wide cFDR values were also tested for enrichment in 9,711 gene sets included in the MAGENTA software package (version 2.4, July 2011) and derived from databases such as Gene Ontology (GO, http://geneontology.org/ ), Kyoto Encyclopedia of Genes and Genomes (KEGG, http://www.kegg.jp/ ), Protein ANalysis THrough Evolutionary Relationships (PANTHER, http://www.pantherdb.org/ ) and INGENUITY ( http://www.ingenuity.com/ ). SNPs were mapped to genes including 20 kb up- and downstream regions to include regulatory elements. The enrichment cutoff applied in our analysis was based on the 95th percentile of gene scores for all genes in the genome. The null distribution of gene scores for each gene set was based on 10,000 randomly sampled gene sets with equal size. MAGENTA uses a Mann–Whitney rank-sum test to assess gene-set enrichment [39] . Data availability All data used in this study are publically available and can be accessed via the studies cited in the text. Other data are available from the authors upon reasonable request. How to cite this article : McLaughlin, R. L. et al . Genetic correlation between amyotrophic lateral sclerosis and schizophrenia. Nat. Commun . 8 , 14774 doi: 10.1038/ncomms14774 (2017). Publisher’s note: Springer Nature remains neutral with regard to jurisdictional claims in published maps and institutional affiliations.